A mutation in the enzyme monoamine oxidase explains part of theAstyanaxcavefish behavioural syndrome We use Astyanax mexicanus , a single species with surface-dwelling forms (SF) and blind de-pigmented cave forms (CF), to study mechanisms underlying the evolution of brain and behaviour. In CF, the origin of changes in complex motivated behaviours (social, feeding, sleeping, exploratory) is unknown. Here we find a hyper-aminergic phenotype in CF brains, including high levels and neurotransmission indexes for serotonin, dopamine and noradrenaline, and low monoamine oxidase (MAO) activity. Although MAO expression is unchanged in CF, a pro106leu mutation is identified in the MAO coding sequence. This mutation is responsible for low MAO activity and high serotonin neurotransmission index in CF brains. We find the same mutated allele in several natural CF populations, some being independently evolved. Such occurrence of the same allele in several caves may suggest that low MAO activity is advantageous for cave life. These results provide a genetic basis for several aspects of the cavefish ‘behavioural syndrome’. The fish species Astyanax mexicanus exists under two forms: river-dwelling morphs and cave-adapted morphs which live in the San Luis Potosi region in Mexico and which are blind and de-pigmented [1] . Cavefish are distributed in 29 caves and correspond to at least two distinct lineages, ‘old’ and ‘new’ [2] , [3] , [4] , [5] , [6] among which individual cave populations have evolved independently at least five times [7] , [8] . These two Astyanax morphs are advantageously used in comparative and evolutionary studies [9] , [10] , [11] . Indeed, during the approximately 1 MY since they evolved from their river-dwelling and sighted ancestors [8] , cavefish have evolved a number of morphological, physiological and behavioural traits, most likely in adaptation to the darkness of their subterranean habitat. In particular, Astyanax cave morphs have lost their eyes and their pigmentation, and they have also lost sleep [12] , [13] , schooling [14] , [15] and hierarchical aggressive behaviour [16] , [17] , [18] . On the other hand, they have gained adaptive behaviours such as attraction to vibrations [19] , increased exploratory [20] , [21] , [22] , [23] , [24] and food searching behaviour [17] , and a special feeding posture [25] , [26] . This is sometimes referred to as ‘the cavefish behavioural syndrome’. Developmental evolution of specific neural circuits is involved in some of these behavioural changes: an increase in the number of serotonin neurons in the cave forms (CF) hypothalamus was shown responsible for their persistent food searching behaviour [17] , and an increase in the number of their head neuromasts is responsible for the emergence of the vibration attraction behaviour [27] . But the origin of most changes in complex motivated behaviours is unknown. The broad neuromodulatory control exerted by monoamines in vertebrate brains explains why they have been implicated in a variety of functions and processes (attention and arousal (Noradrenaline, NA), defence and anxiety (dopamine, DA; serotonin, 5-HT), stress and emotions (DA, NA, 5-HT), reward (DA), mood (5-HT), appetite and energy expenditure, sleep/wakefulness (5-HT, NA, Melatonin), motor control (DA, 5-HT), or cognition) and why their deregulation is involved in various pathologies. In fish, monoaminergic systems have recently attracted interest, partly because the zebrafish ( Danio rerio ) appears as a suitable laboratory animal to model some aspects of complex behaviours [28] and to study and screen neuroactive molecules [29] , [30] . Indeed, monoaminergic systems are globally well conserved and seem to serve the same types of functions in fish and mammals, with some anatomical and genetic exceptions [31] , [32] . These include the presence of 5-HT and DA cell bodies in the fish forebrain (5-HT [17] , [33] , [34] , [35] , [36] , [37] ; DA [32] , [38] , [39] , [40] , [41] , [42] ). Also, there are two tyrosine hydroxylases ( THs ) [43] , two tryptophan hydroxylases ( TPH ) [44] , and two putative COMT genes [32] in zebrafish (see Fig. 1a ). Conversely, and this is a notable exception, there is only one monoamine oxidase ( MAO ) gene in all teleosts examined so far (zebrafish, carp, trout and rainbow trout, pike and catfish [45] , [46] , [47] , [48] , [49] , [50] ), whereas two forms of this enzyme, MAO-A and MAO-B, are classically described and studied in mammals [51] , [52] , [53] , [54] . 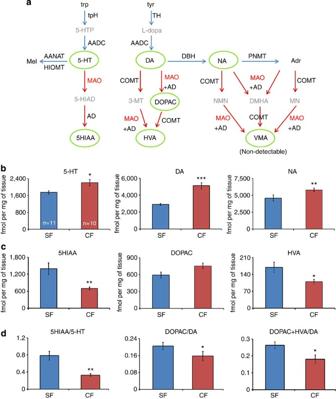Figure 1: HPLC measurements of monoamines and metabolites inAstyanaxSF and Pachón CF. (a) Schema of the principal synthesis and degradation pathways for monoamines. Emphasis is given on the compounds and enzymes studied (MAO in red). A green circle indicates the molecules analysed by HPLC. (b,c) HPLC measurements of indicated monoamines (b) and metabolites (c) in whole brains of SF (blue) and CF (red). VMA was undetectable (<50 fmol per mg tissue). (d) Calculated metabolite/monoamine ratios in SF (blue) and CF (red). Values are indicated as mean±s.e.m. Mann–Whitney statistical tests were used and performed with the Statview software. *P<0.05, **P<0.01 and ***P<0.001. Figure 1: HPLC measurements of monoamines and metabolites in Astyanax SF and Pachón CF. ( a ) Schema of the principal synthesis and degradation pathways for monoamines. Emphasis is given on the compounds and enzymes studied (MAO in red). A green circle indicates the molecules analysed by HPLC. ( b , c ) HPLC measurements of indicated monoamines ( b ) and metabolites ( c ) in whole brains of SF (blue) and CF (red). VMA was undetectable (<50 fmol per mg tissue). ( d ) Calculated metabolite/monoamine ratios in SF (blue) and CF (red). Values are indicated as mean±s.e.m. Mann–Whitney statistical tests were used and performed with the Statview software. * P <0.05, ** P <0.01 and *** P <0.001. Full size image Here we investigate differences in brain aminergic neurochemistry in surface and cave Astyanax . We find high neurotransmission indexes for 5-HT, DA and NA, and low MAO activity in cavefish brains. We then identify a mutation in the MAO coding sequence of cavefish, the same allele being present in several independently evolved natural populations of cavefish. We propose that this mutation could underlie some of the behavioural peculiarities of cavefish, including loss of aggressiveness, absence of schooling and persistent foraging behaviour. Aminergic neurochemistry of surface and cavefish brains The levels of 5-HT, NA, DA and their metabolites were measured by high-performance liquid chromatography (HPLC) in the brains of 3- to 4-month-old surface-dwelling forms (SF) and CF juveniles of the Pachón cave. The synthesis and degradation pathways for the studied monoamines are schematized in Fig. 1a . During dissections, two main parts of the brains were separated through a cut at the level of the midbrain/hindbrain junction ( Supplementary Fig. 1a ) but for simplification the results are given in Fig. 1 as total brain amounts. Levels of 5-HT, DA and NA were significantly higher in Pachón brains, particularly in the anterior part ( Supplementary Fig. 1b ). These globally higher levels of the ‘primary’ monoamines found in Pachón brains are not due to a differential activity of their biosynthetic enzymes, as tyrosine hydroxylase (TH) and tryptophan hydroxylase (TPH) enzymatic activities are identical in brain extracts of the two morphs (TH: SF: 0.357±0.04 and CF: 0.395±0.06, P =0.188. TPH: SF: 0.419±0.02 and CF: 0.387±0.01, P =0.528; both activities expressed in nmoles per mg protein per hour, n =8 each. Mann–Whitney test. Throughout text, values are given as mean±s.e.m.). We next compared the levels of monoamine metabolites ( Fig. 1c ). The intermediate DA metabolite DOPAC showed similar levels in SF and CF, whereas the final DA metabolite HVA was found at lower levels in CF brains. The levels of the 5-HT metabolite 5HIAA were twice lower in CF brains ( Fig. 1c ). This suggests that the MAO enzyme has differential activities in SF and Pachón. The ‘intensity’ index of a neurotransmitter system can be assessed through its metabolite/neurotransmitter ratio: the higher this ratio, the stronger the catabolic activity, the weaker the neurotransmission index. We therefore expressed HPLC results as metabolite/neurotransmitter ratios ( Fig. 1d ). All three ratios 5HIAA/5-HT, DOPAC/DA and DOPAC+HVA/DA were significantly lower in Pachón brains than in SF, suggesting stronger 5-HT and DA neurotransmissions in Pachón. This was particularly true for the anterior part of the brain ( Supplementary Fig. 1d ). These indexes being dependent on the activity of the MAO enzyme further suggest a differential activity of this degrading enzyme in the two morphs. We thus compared MAO enzymatic activity in the brains of the two Astyanax morphs. Importantly and contrary to mammals, all teleosts tested so far have only one MAO (also true for Astyanax , see next paragraphs). Thus, we tested MAO activity in vitro on 3-month-old SF and Pachón total brain extracts on three different substrates that are widely used in the literature to assay mammalian MAO-A and/or MAO-B activities: 5-HT, β-phenylethylamine and tyramine. In all three assays, MAO activity was detected, therefore showing both MAO-A- and MAO-B-like properties. Moreover, with all three substrates, MAO activity was about twice lower in Pachón brains ( Fig. 2a ). In parallel, MAO activity was assessed in situ in larval brains using tyramine as substrate, and showed lighter staining in Pachón brains ( Fig. 2b,c ). 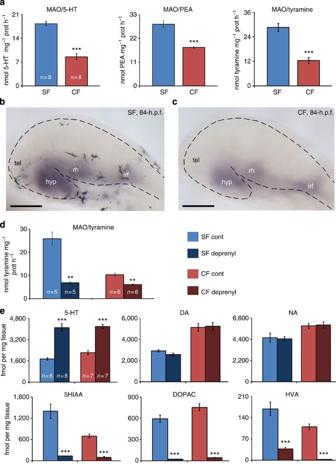Figure 2: MAO activity inAstyanaxSF and Pachón CF. (a) MAO enzymatic activity measurements using indicated substrates in whole brains of SF (blue) and CF (red). PEA, β-phenylethylamine. 5-HT, PEA and tyramine are preferential substrates for mammalian MAO-A, MAO-B or both, respectively. (b,c)In situMAO activity on whole 84-h.p.f. larvae brains pictured on lateral views. Anterior is left and dorsal is up. The intensity of staining is higher in SF brain, suggesting a higher MAO activityin situthat parallels the higher activityin vitro. Scale bar, 200 μm. (d) Effect of deprenyl (10 μM, dark blue and dark red bars) on MAO enzymatic activity in brain extracts from SF and Pachón CF, using tyramine as substrate. (e) Effect of deprenyl (10 μM, dark blue and dark red bars) on amine and metabolite levels in brain extracts from SF and Pachón CF, measured by HPLC. Values are indicated as mean±s.e.m. Mann–Whitney statistical tests were used and performed with the Statview software. **P<0.01 and ***P<0.001. hyp, hypothalamus; irf, internal reticular formation; rh, rhombencephalon; tel, telencephalon. Figure 2: MAO activity in Astyanax SF and Pachón CF. ( a ) MAO enzymatic activity measurements using indicated substrates in whole brains of SF (blue) and CF (red). PEA, β-phenylethylamine. 5-HT, PEA and tyramine are preferential substrates for mammalian MAO-A, MAO-B or both, respectively. ( b , c ) In situ MAO activity on whole 84-h.p.f. larvae brains pictured on lateral views. Anterior is left and dorsal is up. The intensity of staining is higher in SF brain, suggesting a higher MAO activity in situ that parallels the higher activity in vitro . Scale bar, 200 μm. ( d ) Effect of deprenyl (10 μM, dark blue and dark red bars) on MAO enzymatic activity in brain extracts from SF and Pachón CF, using tyramine as substrate. ( e ) Effect of deprenyl (10 μM, dark blue and dark red bars) on amine and metabolite levels in brain extracts from SF and Pachón CF, measured by HPLC. Values are indicated as mean±s.e.m. Mann–Whitney statistical tests were used and performed with the Statview software. ** P <0.01 and *** P <0.001. hyp, hypothalamus; irf, internal reticular formation; rh, rhombencephalon; tel, telencephalon. Full size image Most of what is currently known on monoamine metabolism in fish comes from the zebrafish model. In this species, MAO is inhibited by both clorgyline and deprenyl [45] (selective mammalian MAO-A and MAO-B inhibitors, respectively) and displays strong affinity for 5-HT but a modest one for DA, so that MAO inhibition by deprenyl strongly increases 5-HT but not DA and NA levels [37] . We therefore better characterized MAO properties in our model, using deprenyl. Astyanax MAO activity in brain extracts was strongly affected after a treatment with deprenyl (10 μM) in both SF and CF ( Fig. 2d ). Moreover, and as expected, after MAO inhibition, 5-HT levels were strongly increased, whereas 5HIAA levels were strongly decreased in both SF and CF brains ( Fig. 2e ). DOPAC and HVA were also diminished after deprenyl, but DA levels were unaffected ( Fig. 2e ), suggesting that DA is a poor MAO substrate. Finally, NA levels were also unaffected by deprenyl ( Fig. 2e ). Combined to our finding of undetectable VMA levels in Astyanax brains ( Fig. 1a ), this suggests that NA is not degraded by MAO in this fish. Importantly, SF and CF MAO enzymatic activity and biochemical profiles were affected identically by deprenyl ( Fig. 2d,e ). Taken altogether, these data show that low MAO activity in the CF brains explains well the high 5-HT and low 5HIAA levels, and the CF ‘hyper-serotonergic’ biochemical profile. We next explored two main and non-exclusive hypotheses, that is, a change in MAO expression and/or a change in MAO sequence in Pachón. MAO expression in surface fish and Pachón cavefish We cloned a 635-bp fragment of Astyanax SF and Pachón CF MAO complementary DNA (cDNA). After phylogenetic analysis, Astyanax MAO grouped consistently with sequences from other teleosts ( Fig. 3a and Supplementary Fig. 2 ). The deduced Astyanax SF amino-acid sequence is 95% identical to zebrafish, and 79–78% identical to mouse MAO-A and MAO-B, respectively. Checking in the preliminary contigs assembly of the A. mexicanus Pachón genome (GenBank Assembly accession code GCA_000372685.1 ) further confirmed that there is only one form of the enzyme, like in other teleosts. The cloned fragment was used as a probe to compare the spatio-temporal MAO expression patterns in larval brains of SF and CF ( Fig. 3b,c ). The onset of MAO expression in Astyanax was before 36-h.p.f. MAO transcripts were detected with similar signal intensities in SF and CF larvae of 36–60-h.p.f., throughout the diencephalon and hypothalamus, and in discrete groups of cells in the hindbrain corresponding to raphe, locus coeruleus and internal reticular formation neurons at later stages. MAO expression was interpreted with respect to the distribution of TH-expressing cells (corresponding to DA and NA groups) and 5-HT cells ( Fig. 3d,e ). All the first MAO -expressing cells in the brain correspond to 5-HT cells and to a subset of DA and NA cells, and are located in those regions with high in situ MAO activity (compare with Fig. 2b,c ). Because in situ hybridization is not a quantitative method, we next performed semiquantitative PCR to check for potential differences in MAO mRNA expression levels, using α-actin as a control ( Fig. 3f ). MAO cDNA amplification from reverse-transcribed mRNA of 1-week-old larval heads was identical in SF and Pachón. Finally, MAO protein concentrations, assessed by measuring the binding of two selective mammalian MAO-A and MAO-B inhibitors, were identical in SF and Pachón brains ( Fig. 3g ). Thus the onset, the pattern and the levels of MAO mRNA and protein expression are identical in the brains of the two Astyanax morphs. 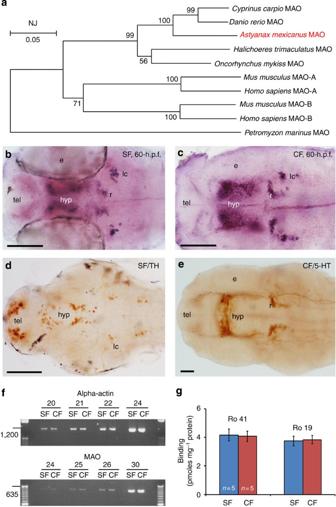Figure 3:MAOexpression inAstyanaxSF and Pachón CF. (a) Phylogenetic tree (neighbor joining, NJ) showing the relationships betweenAstyanaxand other vertebrateMAOsequences. All teleosts have only one form of the enzyme. A duplication occurred in the amniote lineage. Bootstrap values are indicated.Cyprinus carpio: carp.Danio rerio: zebrafish.Halichoeres trimaculatus: threespot wrasse.Oncorhynchus mykiss: trout.Petromyzon marinus: marine lamprey (outgroup). (b,c)In situhybridization forMAOmRNA, ventral views of dissected brains of 60-h.p.f. SF and CF larvae. Anterior is left. Scale bar, 100 μm. (d) Immunohistochemistry for TH, ventral view of a 60-h.p.f. SF dissected brain (eyes were removed). Scale bar, 100 μm. (e) Immunohistochemistry for 5-HT; ventral view of a 36-h.p.f. CF dissected brain. Scale bar, 100 μm. (f) Semiquantitative RT–PCR assessment forα-actin(top) andMAO(bottom) mRNA expression levels. After calibration withα-actin, the bands corresponding toMAOamplification appear at the same PCR cycle in SF and CF samples. (g) Binding assays to measure MAO protein concentrations, using the indicated ligands, in whole brains of SF (blue) and CF (red). tel, telencephalon; hyp, hypothalamus; rh, rhombencephalon; irf, internal reticular formation; e, eye; r, raphe nucleus; lc, locus coeruleus. Values are indicated as mean±s.e.m. Mann–Whitney statistical tests were used and performed with the Statview software. Significance was set atP<0.05. Figure 3: MAO expression in Astyanax SF and Pachón CF. ( a ) Phylogenetic tree (neighbor joining, NJ) showing the relationships between Astyanax and other vertebrate MAO sequences. All teleosts have only one form of the enzyme. A duplication occurred in the amniote lineage. Bootstrap values are indicated. Cyprinus carpio : carp. Danio rerio : zebrafish. Halichoeres trimaculatus : threespot wrasse. Oncorhynchus mykiss : trout. Petromyzon marinus : marine lamprey (outgroup). ( b , c ) In situ hybridization for MAO mRNA, ventral views of dissected brains of 60-h.p.f. SF and CF larvae. Anterior is left. Scale bar, 100 μm. ( d ) Immunohistochemistry for TH, ventral view of a 60-h.p.f. SF dissected brain (eyes were removed). Scale bar, 100 μm. ( e ) Immunohistochemistry for 5-HT; ventral view of a 36-h.p.f. CF dissected brain. Scale bar, 100 μm. ( f ) Semiquantitative RT–PCR assessment for α-actin (top) and MAO (bottom) mRNA expression levels. After calibration with α-actin , the bands corresponding to MAO amplification appear at the same PCR cycle in SF and CF samples. ( g ) Binding assays to measure MAO protein concentrations, using the indicated ligands, in whole brains of SF (blue) and CF (red). tel, telencephalon; hyp, hypothalamus; rh, rhombencephalon; irf, internal reticular formation; e, eye; r, raphe nucleus; lc, locus coeruleus. Values are indicated as mean±s.e.m. Mann–Whitney statistical tests were used and performed with the Statview software. Significance was set at P <0.05. Full size image A mutation in the Pachón cavefish MAO sequence One significant coding sequence difference between Pachón CF and SF MAO was detected: a Proline (Pro) to Leucine (Leu) substitution due to a point mutation (CCG>CTG) was observed in 5/5 independent clones of Pachón CF MAO cDNA at position 106, suggesting that the amino-acid change is fixed in our lab-bred Pachón population ( Fig. 4a , red arrow and Supplementary Fig. 3a ). This substitution is located in a highly conserved region and at a position where a leucine is found in SF and in all other vertebrate species. Such a substitution is considered as ‘radical’, the two amino acids having different physico-chemical properties. Moreover, six polymorphic sites are found in Pachón MAO ; each in one of the five independent clones of Pachón MAO sequenced ( Supplementary Fig. 3a , black arrows). The rest of the sequence, including the highly conserved NAD(P)-binding Rossmann-like domain (catalytic domain; Pfam13450) is identical in the two morphs. 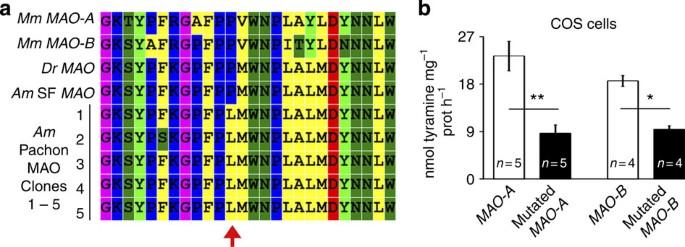Figure 4: AMAOmutation in cave-dwellingAstyanax mexicanus. (a) Alignment of amino acids in the region of interest between mammalianMAO-A/B, zebrafishMAO, andAstyanaxSF and PachónMAOs. A red arrow indicates the fixed substitution (Pro106Leu) in Pachón CFMAO.Mm,Mus musculus;Dr,Danio rerio;Am,Astyanax mexicanus.(b) MAO enzymatic activity, measured using tyramine as substrate, on COS-7 cells transfected with pro>leu mutated mouseMAO-AandMAO-B. Mann-Whitney statistical tests were used and performed with the Statview software. *P<0.05, **P<0.01. Figure 4: A MAO mutation in cave-dwelling Astyanax mexicanus . ( a ) Alignment of amino acids in the region of interest between mammalian MAO-A/B , zebrafish MAO , and Astyanax SF and Pachón MAOs . A red arrow indicates the fixed substitution (Pro106Leu) in Pachón CF MAO . Mm , Mus musculus ; Dr , Danio rerio ; Am , Astyanax mexicanus. ( b ) MAO enzymatic activity, measured using tyramine as substrate, on COS-7 cells transfected with pro>leu mutated mouse MAO-A and MAO-B . Mann-Whitney statistical tests were used and performed with the Statview software. * P <0.05, ** P <0.01. Full size image To test whether Pro106Leu in Pachón MAO is responsible for its decreased enzymatic activity, we performed site-directed mutagenesis on mouse MAO-A and MAO-B to mimic the CF Pro>Leu substitution. In COS-7 cells transfected with either form of mutated mammalian MAO , MAO activity was twice lower than in control-transfected cells ( Fig. 4b ). This shows that Pro106Leu significantly affects the function of the enzyme. Of note, comparing results from SF/Pachón and from control/mutated-transfected COS shows that the loss of activity is proportionally similar in both cases ( P =0.3082, Mann–Whitney test). These data suggest that Pro106Leu is sufficient to explain the difference of MAO activity observed between SF and Pachón CF. Pro106Leu MAO mutation in natural cavefish populations We next sought to check whether the Pro106Leu mutation was also present in wild-caught individuals of the Pachón cave, and possibly of other caves. PCR was performed on genomic DNA extracted from fin-clips to amplify MAO exon4 (which encodes the amino-acid position 106). Exon4 was sequenced in wild-caught individuals of Pachón, Los Sabinos, Tinaja, Rio Subterráneo and Molino caves, as well as in SF caught in Rio Valles near Micos ( Fig. 5a ). Wild-caught SF and Pachón had a proline (homozygotes, n =5) and a leucine (homozygotes, n =4) at position 106, respectively, and were therefore identical to lab-raised populations ( Supplementary Fig. 3b ). Tinaja ( n =3) and Los Sabinos ( n =3) individuals also presented the Pachón leu 106 allele, due to the same C>T mutation, either as homozygotes or as heterozygotes ( Fig. 5a,b and Table 1 ). Conversely, the leu 106 allele was not found in individuals of the Rio Subterráneo ( n =8) or Molino ( n =7) populations, proposed to derive from a ‘new’ invasion event [7] . 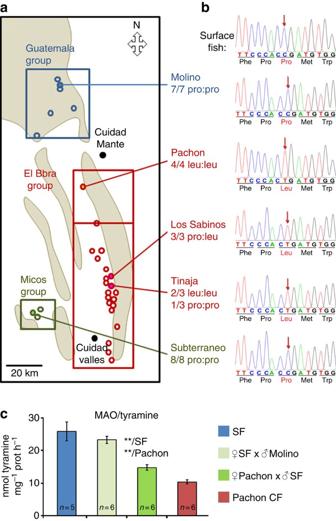Figure 5: Distribution ofMAOalleles in the wild. (a) Distribution ofMAOalleles in Mexican caves on a map redrawn and adapted from refs7,10. Each circle indicates a cave hosting cavefish. The cavefish inhabiting the ‘El Abra group’ originate from an ancient colonization and can further be subdivided into two independent colonization events, while those inhabiting caves from Guatemala and Micos group are supposed to be more recent7. Caves from which fin-clips have been analysed are indicated, with their corresponding allele distribution. (b) Sequence chromatograms centred aroundMAOamino-acid 106, showing that Pachón, Tinaja and Los Sabinos share the exact same allele for leu106. Also note that SF, Molino and Subterraneo, as well as those individuals with a pro106allele in Tinaja and Los Sabinos, share the same proline codon. (c) MAO enzymatic activity, measured using tyramine as substrate, in brain extracts from F1 hybrid individuals obtained after crosses between a Pachón female and a SF male (Pa × SF), or between a SF female and a Molino male (SF × Mo). Values are indicated as mean±s.e.m. Mann–Whitney statistical tests were used and performed with the Statview software. **P<0.01. Figure 5: Distribution of MAO alleles in the wild. ( a ) Distribution of MAO alleles in Mexican caves on a map redrawn and adapted from refs 7 , 10 . Each circle indicates a cave hosting cavefish. The cavefish inhabiting the ‘El Abra group’ originate from an ancient colonization and can further be subdivided into two independent colonization events, while those inhabiting caves from Guatemala and Micos group are supposed to be more recent [7] . Caves from which fin-clips have been analysed are indicated, with their corresponding allele distribution. ( b ) Sequence chromatograms centred around MAO amino-acid 106, showing that Pachón, Tinaja and Los Sabinos share the exact same allele for leu 106 . Also note that SF, Molino and Subterraneo, as well as those individuals with a pro 106 allele in Tinaja and Los Sabinos, share the same proline codon. ( c ) MAO enzymatic activity, measured using tyramine as substrate, in brain extracts from F1 hybrid individuals obtained after crosses between a Pachón female and a SF male (Pa × SF), or between a SF female and a Molino male (SF × Mo). Values are indicated as mean±s.e.m. Mann–Whitney statistical tests were used and performed with the Statview software. ** P <0.01. Full size image Table 1 Distribution of MAO alleles in lab-raised and wild animals of the studied caves. Full size table MAO amino-acid 106 position and enzymatic activity Finally, using F1 hybrids between Astyanax morphs with known genotypes, we sought to test directly the effect of the amino-acid 106 position on the enzymatic activity of the MAO enzyme. Thus, MAO activity was measured in the brains of F1 hybrids resulting from a cross between a Pachón female and a SF male (Pa × SF; therefore leu:pro heterozygotes at position 106) and in F1 hybrids resulting from a cross between a SF female and a Molino male (SF × Mo; therefore pro:pro homozygotes at position 106). In SF × Mo (pro:pro), MAO activity was identical to SF, while in Pa × SF (leu:pro) MAO activity was lower than in SF but higher than in Pachón ( Fig. 5c ). These data are consistent with COS-7 cells experiments and suggest a good correlation between MAO genotype (aa106) and phenotype (enzymatic activity). To our knowledge, this report is one of the first examining in depth the monoaminergic biochemical profile in a teleost brain. In our model species Astyanax , some features were strikingly different from what is largely reported in mammals including humans. First, the levels of the final metabolite VMA were undetectable, suggesting that MAO and COMT are not actively degrading NA. Second, deprenyl treatment did not affect DA and NA levels, delineating these amines are poor MAO substrates, like in zebrafish [37] . Finally, like in other teleosts, there is only one form of the MAO enzyme, which effectively de-aminates mammalian MAO-A- or MAO-B-specific substrates, therefore ‘recapitulating’ MAO-A+B types of activities. However, the presence of a single MAO in the catabolism pathway of the monoamines probably imposes some peculiarities on these neurotransmitter systems. An important consequence is that in Astyanax (and probably in other fishes as well) the deprenyl-dependent behaviours may be attributed mainly to the serotonergic system. We report a global hyper-monoaminergic phenotype in CF: neurotransmitter levels are higher and their metabolite/neurotransmitter ratios are lower in CF brains, highlighting a stronger neurotransmission index. Concerning 5-HT, the pro106leu mutation probably plays a major role. We have also previously reported a difference in the size of the PVa hypothalamic nucleus, which is larger and contains more neurons in CF [17] . We can suppose that both decreased MAO activity and higher cell number contribute to the higher 5-HT levels in CF, and it would actually be difficult to discriminate between the two convergent effects. It is also interesting to note that the increased 5-HT levels and increased neurotransmission index were especially robust in the forebrain part of the CF samples, where neuronal nuclei but also extensive fibre projection systems reside. Concerning DA and NA, their elevated levels in CF seem neither due to MAO mutation (as they are poor MAO substrates) nor due to differences in activity of TH and TPH biosynthetic enzymes. Interestingly, a recent study proposed a role for an independent mutation in the gene Oca2 ( Ocular and Cutaneous Albinism 2 ). In fact, a mutation in Oca2 is known to cause albinism in CF [55] , as it stops the melanin biosynthesis pathway at the step of L-tyrosine. As a consequence, L-tyrosine, which is also the precursor of DA and NA, is not metabolized in CF. Interestingly, Oca2 morpholino knockdown in SF embryos was recently shown to increase both L-tyrosine and DA levels, suggesting that an expanded L-tyrosine pool is available as a precursor for DA in CF [56] . Taken altogether, these data suggest that CF have elevated brain levels of 5-HT and DA (and secondarily NA) caused by two independent mutations in MAO and Oca2 , respectively. The Pro106Leu substitution in the cavefish MAO appears like a partial loss of function mutation. The high number of SNPs surrounding this fixed mutation suggests that this region of the protein is prone to mutations (and maybe rapid evolution) in the cavefish lineage. This corresponds to the ‘molecular evolution’ component of the change in 5-HT transmission in cavefish. On the other hand, the increased number of cells in the hypothalamus appears like a gain-of-function phenotype. We have recently shown that the change of size of this particular nucleus in cavefish is due to early developmental signalling and neurogenesis timing differences during embryogenesis of the two morphs [17] . Such change corresponds to the ‘developmental evolution’ component of the variation in monoamine transmission in cavefish. Strikingly, the loss of function/molecular evolution and the gain-of-function/developmental evolution components of the changes observed in cavefish both contribute to an enhancement of 5-HT neurotransmission. This suggests that the CF hyper-serotonergic phenotype could be adaptive for life in cave environment. We have studied monoamines in Astyanax SF and CF brains because these neurotransmitter systems seemed relevant to the known behavioural differences that exist between the two morphs. Some of the well-supported functional correlations are discussed thereafter ( Fig. 6 ). First, the MAO mutation and decreased MAO activity in CF may constitute part of the molecular basis for changes in ‘social’ behaviours in cavefish, including their loss of aggressiveness [17] , [57] and schooling [14] behaviours. Accordingly, deprenyl-treated SF show reduced aggressiveness [17] and reduced schooling [14] , whereas deprenyl-treated CF show no change in these behaviours. In fact, in SF, the aggressiveness (measured as attacks between individuals in behavioural tests) corresponds to the establishment of hierarchy between fish, and this behaviour is driven by 5-HT neurons of the raphe nucleus in the hindbrain [17] . Moreover, this hierarchical aggressiveness is inversely correlated with the intensity of 5-HT neurotransmission. Evidence for this statement comes from deprenyl treatment that strongly decrease the number of attacks between two SF, and from HPLC measurements of 5-HT content in the raphe nucleus that is much lower in dominant than in subordinate SF individuals [17] . We therefore proposed that dominant aggressiveness in SF results from an experience-dependent downregulation of 5-HT content in the raphe. However, the loss of aggressiveness in Pachón CF remained unexplained mechanistically, and was hypothesized to result from an inability of CF to downregulate their raphe 5-HT levels. The present finding of a mutation in the MAO that affects its enzymatic activity, and that condemns CF to have high brain 5-HT levels (including in the raphe) now provides a molecular basis to the hypothesis. Concerning schooling [14] , [15] , part of its loss in CF is due to the fact that schooling is dependent on vision (cavefish are blind), but part of it is not. In addition, schooling in SF is abolished after deprenyl treatment [14] . It was therefore hypothesized that brain monoamines were involved in the control of schooling in SF. Our present data narrow down and identify the candidate neurotransmitter as serotonin, as due to the fish-specific condition only 5-HT levels (but not DA or NA levels) are affected by deprenyl. Again, the present finding of a MAO mutation that affects its enzymatic activity and that confers CF with high brain 5-HT levels provides a molecular basis to the experimental evidence for the loss of schooling. Of note, Kowalko et al. [14] used Tinaja (not Pachón) as Astyanax cavefish population in their study. Here we show that the leu 106 allele is also present in the Tinaja population. Finally, we have previously proposed that the loss of aggressiveness in cavefish is related to a general loss of social or collective behaviours during their evolution in subterranean environment [57] . Therefore, the loss of aggressiveness and the loss of schooling could be somehow ‘linked’, both resulting from the MAO mutation and from the ‘hyper-serotonergic’ phenotype. However, the exact 5-HT neuronal group that participates in the control of schooling is not known. 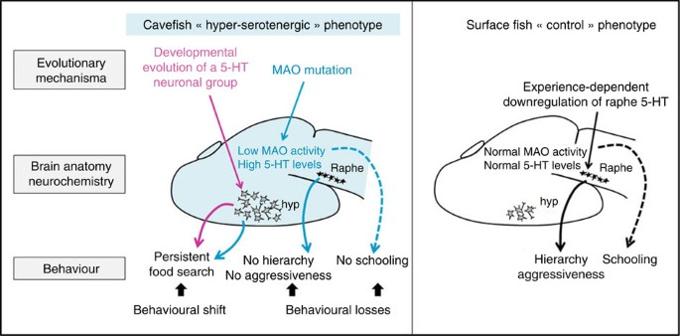Figure 6:MAOand serotonergic phenotypes in Pachón cavefish. A schematic drawing puts the present results in the bibliographical context of what was previously established on behavioural evolution in cavefish. Only the serotonergic system is shown. Top, evolutionary mechanisms. Middle, brain anatomy and neurochemistry. Bottom, behavioural outcome. Three types of cavefish behavioural modifications (food search, loss of aggressiveness and loss of schooling) can be attributed to 5-HT neurotransmission, based on their sensitivity to deprenyl. In red, developmental evolution of a neuronal 5-HT group of the anterior hypothalamus contributes to higher 5-HT content in the forebrain of the Pachón CF. This process is dependent on Sonic Hedgehog signalling during early embryogenesis and leads to a cavefish-specific behavioural phenotype consisting in persistent foraging17,57. In blue, theMAOmutation leads to low MAO activity and high 5-HT content throughout the CF brain. This impacts raphe-driven aggressive behaviour (plain arrows), as cavefish are unable to downregulate their raphe 5-HT levels like dominant SF do17. This probably also impacts schooling behaviour, shown to be deprenyl-dependent14. The dashed line relationship between brain 5-HT content and schooling is solely to indicate that no specific brain region has been identified yet to drive this behaviour. Figure 6: MAO and serotonergic phenotypes in Pachón cavefish. A schematic drawing puts the present results in the bibliographical context of what was previously established on behavioural evolution in cavefish. Only the serotonergic system is shown. Top, evolutionary mechanisms. Middle, brain anatomy and neurochemistry. Bottom, behavioural outcome. Three types of cavefish behavioural modifications (food search, loss of aggressiveness and loss of schooling) can be attributed to 5-HT neurotransmission, based on their sensitivity to deprenyl. In red, developmental evolution of a neuronal 5-HT group of the anterior hypothalamus contributes to higher 5-HT content in the forebrain of the Pachón CF. This process is dependent on Sonic Hedgehog signalling during early embryogenesis and leads to a cavefish-specific behavioural phenotype consisting in persistent foraging [17] , [57] . In blue, the MAO mutation leads to low MAO activity and high 5-HT content throughout the CF brain. This impacts raphe-driven aggressive behaviour (plain arrows), as cavefish are unable to downregulate their raphe 5-HT levels like dominant SF do [17] . This probably also impacts schooling behaviour, shown to be deprenyl-dependent [14] . The dashed line relationship between brain 5-HT content and schooling is solely to indicate that no specific brain region has been identified yet to drive this behaviour. Full size image Second, the MAO-dependent high 5-HT neurotransmission index is also relevant to CF-increased foraging behaviour [17] , [57] and behavioural drive for food (hypothesis in ref. 58 ). Accordingly, deprenyl-treated CF show persistent foraging [17] . DA may as well play a role in what could be described as a sort of ‘addiction’ to food in CF. Third, elevated NA brain levels in CF may be related to their reported loss of sleep [13] . Consistently, a blockade of β1-adrenergic receptors rescues sleep in CF [12] , indeed involving the NA system in this striking behavioural peculiarity. And finally, cavefish swim constantly and longer distances than SF, but this enhanced locomotor activity is unaffected by deprenyl [17] , ruling out an involvement of the 5-HT system. In this case, DA or NA neurotransmission could be involved. We have found the same leu 106 allele in several caves of the El Abra group of caves. As Los Sabinos/Tinaja and Pachón populations are proposed to derive from independent events of the ‘old’ invasion of caves [7] , two hypotheses can be proposed: either the leu 106 allele has been selected (at least twice) in independent caves, probably from standing genetic variation in the surface-dwelling ancestral population; or the leu 106 allele has spread from one of the El Abra caves to the others through cross-hybridizations in the complex underground water system and gene flow between populations. In any case, and again, it suggests that low MAO activity is advantageous for cave life. In humans, MAO-A/B sequences seem very constrained as only two point mutations in the coding sequence of MAO-A have been described in patients with intellectual disability and impulsive, violent behaviour [59] , [60] . The cavefish aminergic condition, including high neurotransmission indexes and a mutation in their MAO enzyme, would probably be considered strongly pathological in humans [61] , yet they thrive in their caves since about one million years. Fish Laboratory stocks of A. mexicanus surface fish and cavefish (Pachón population) were obtained in 2004–2006 from the Jeffery laboratory at the University of Maryland, College Park, MD, USA and were since then bred in our local facility. Fish were maintained at 23–26 °C on 12:12-h light: dark cycle and they were fed twice a day with dry and living food. The fry were raised in Petri dishes and fed with 2-day-old artemia after opening of the mouth [62] . Animals were treated according to the French and European regulations for handling of animals in research. SR’s authorization for use of animals in research is number 91–116, and Paris Centre-Sud Ethic Committee authorization numbers are 2012-0054 and -0056. Fin-clips from wild-caught animals were collected under the auspices of Mexican permit 02241/13 delivered to SR by Secretaria de Medio Ambiente y Recursos Naturales. HPLC HPLC assays were performed on fresh tissue. Three- to five-month-old juvenile fish were euthanized by immersion in ice-cold water for 1 min, weighed, measured and sexed. Brains were rapidly dissected out on ice and cut in two parts at the level of the midbrain/hindbrain junction: the anterior part which, in fish, contains the 5-HT hypothalamic neurons and the DA telencephalic, hypothalamic and posterior tuberculum neuronal groups and the posterior part which contains the 5-HT raphe hindbrain neurons and the locus coeruleus and rhombencephalic NA neurons, which are similar to mammals. Samples were immersed in hydrochloric acid (10 −3 M), weighed and frozen at −80 °C. Before analysis, brains were crushed and centrifuged at 22,000 g for 20 min at 5 °C. The supernatants were collected and filtered through a 10-kDa membrane (Nanosep, Pall) by centrifugation at 7,000 g . Then, a 20-μl aliquot of sample was analysed for serotonin (5-HT) by fluorometric detection. The amounts of catecholamines (dopamine/DA, noradrenalin/NA) and their metabolites (DOPAC, HVA) as well as the 5-HT metabolite 5HIAA were measured by electrochemical detection on a serial array of coulometric flow-through graphite electrodes (CoulArray, ESA). The analysis, data reduction and peak identification were fully automated. Results were expressed as fentomoles per mg of fresh tissue. Deprenyl treatments We used R-deprenyl hydrochloride (Sigma Aldrich) dissolved in tank water. Deprenyl (10 μM) was added during 5 h before the sacrifice of the animals. MAO activity In vitro : MAO (EC.1.4.3.4.) enzymatic activities were determined on whole-brain homogenates or on cell homogenates (after thawing, tissues or cells were homogenized in 5 volumes of 0.1 M potassium phosphate buffer, pH 7.40, using all glass homogenizers, Potter–Elvehjem) by a radioenzymatic assay using either [ 14 C]-5-HT creatinine sulphate (1.96 GBq mmol −1 , Amersham GE Healthcare, Saclay, France, final concentration 20 μM), or [ 14 C]-β-phenylethylamine (2.07 GBq mmol −1 , Amersham GE Healthcare, Saclay, France, final concentration 20 μM), or [1, 14 C]-tyramine hydrochloride (1.85 Bq mmol −1 , final concentration 20 μM) as substrates. In brief, 20-μl aliquots of the homogenates were pre-incubated (possibly with an inhibitor) in a total volume of 220 μl at 37 °C for 30 min. At the end of the pre-incubation period, the enzyme reaction was started by addition of 80 μl of one MAO substrate and the incubation continued for 10 min at 37 °C. Then, the reaction was stopped by addition of 200 μl of 2 N HCl, and the deaminated metabolites were extracted by vigorous shaking for 10 min with 5 ml of diethylether (5-HT extraction) or n -heptane (PEA extraction) or anisole (tyramine extraction). After centrifugation (1,000 g ; 30 s) the water phase was frozen in dry ice and the organic layer poured into plastic vials containing 5 ml of scintillation cocktail. Finally, the radioactivity was determined in a scintillation spectrometer. Reaction mixtures as described above, but lacking the homogenate, served as blanks. In our experimental conditions, the enzymatic reaction was linear with time and homogenate concentration. In situ : MAO enzymatic activities were determined in situ on whole larvae. After euthanasia on ice, larvae were frozen on nitrogen and placed in a water bath at 37 °C for 30 min. They were pre-incubated for 30 min in a solution consisting of 1% dimethylsulphoxide (Sigma), 10% of Triton X100 and 10% Tween20 dissolved in 0.05 M Tris-HCL buffer (pH 7.6). The labelling occurred after several hours in the reaction solution consisting of diaminobenzidine tetrachloride (Sigma Aldrich tablets), horseradish peroxidase (ABC kit, Universal Vectastain Kit PK6200), 6 mg ml −1 of nickel ammonium sulphate (Nakarai Chemic LS) and 1 mg ml −1 of tyramine hydrochloride (Sigma), dissolved in 1 ml of 0.05 M Tris–HCl buffer (pH 7.6). MAO protein MAO protein concentration was assessed by measuring the binding of [3H]-Ro 19–6327 [N-(2-aminoethyl)-5-chloropicolinamide HCl, lazabemide] (0.96 TBq mmol −1 , Amersham GE Healthcare, Saclay, France) and [3H]-Ro 41–1049 (0.31 TBq mmol −1 , Amersham GE Healthcare), two selective inhibitors of mammalian MAO-B and MAO-A respectively, to SF and Pachón brains Both ligands gave significant bindings on Astyanax brain samples. A buffer solution (pH=7.40) containing 50 mM Tris, 120 mM NaCl, 1 mM MgCl 2 , 5 mM KCl and 0.5 mM EGTA was used in all experiments. Both radioligands were used at 15 nM final concentration. Incubations were performed for 60 min at 37 °C ([ 3 H]-Ro 41–1049) and for 90 min at 22 °C ( 3 [H]-Ro 19–6327) followed by a 30 s+30 s+1 min wash in cold buffer and a quick dip in cold distilled water. Non-specific binding was determined by incubation in the presence of 1 μM of clorgyline ([ 3 H]-Ro 41–1049) or L-deprenyl ( 3 [H]-Ro 19–6327). Binding quantification was determined by liquid scintillation counting after filtration onto Whatman GF/B glass microfiber disks, which were then soaked in a 2-ml scintillation cocktail overnight with agitation before counting 24 h later (the recovery of this method was consistent since the values of five replicate measurements varied by <5%). MAO cDNA cloning and exon amplification from genomic DNA Total RNA from Pachón CF and SF larvae was reverse transcribed with random primers using AMV reverse transcriptase (Promega). A partial cDNA sequence for MAO (635 bp) was amplified by PCR using the following primers designed on 454 transcriptomic sequence data. MAOF: 5′-GGTCTGAGTGCAGCCAAGCTG-3′. MAOR: 5′-GTGGACCTGGGCGGAGCTTA-3′. PCR products were sub-cloned in TOPO-PCR II vector (Invitrogen) and sequenced. Astyanax MAO sequences were aligned with family members in other species, and phylogenetic trees were constructed with the Neighbour Joining method using MEGA5. Genomic DNA was extracted from fin-clips conserved in ethanol. PCR was then performed on ~20 ng of genomic DNA with the following primers designed to amplify MAO exon4 (150 bp). MAOex4F: 5′-GGGAAATCATATCCATTCAAGGGG-3′. MAOex4R: 5′-CTCCATGCCCATCTTGTCCATAG-3′. PCR products were sub-cloned in TOPO-PCR II vector (Invitrogen) and sequenced. For each individual/fin-clip, a minimum of seven independent clones of exon4 were sequenced to have at least 98.4% chances to detect potential heterozygotes. Semiquantitative PCR In total, 10–20 heads from 1-week-old larvae were immersed in Trizol. Total RNA was extracted as described in the manufacturer’s instructions and reverse transcribed as above. PCR with α-actin primers (actinF: 5′-GGATTCGCTGGAGATGATGCTC-3′; actinR: 5′-CGTCACCTTCACCGTTCCAGT-3′) was used to calibrate for identical amounts of cDNA used as templates for SF and CF. Aliquots from the PCR reaction were removed at successive PCR cycles and loaded on a gel. Immunohistochemistry and in situ hybridization Samples were fixed in (paraformaldehyde 4% in phosphate-buffered saline), gradually dehydrated in methanol and stored at −20 °C. For immunohistochemistry, permeabilization was achieved in phosphate-buffered saline with 1% dimethylsulphoxide and 0.5% Triton, followed by incubation in a rat anti-serotonin primary antibody (Chemicon MAB 352, 1/200) or mouse anti-tyrosine hydroxylase antibody (Vector AbCys, VMA318), followed by secondary biotinylated goat anti-rat antibody (Jackson 112-066-072, 1/500) and biotinylated horse anti-mouse antibody (Vector, BA-2080), respectively. Revelation was performed using an avidin/biotin complex coupled with peroxidase (ABC kit, Universal Vectastain Kit PK6200) and diaminobenzidine (Sigma Aldrich). For in situ hybridization, MAO cDNA (635 bp, see above) was amplified by PCR, and digoxygenin-labelled riboprobes were synthesized from PCR templates. A protocol for automated whole-mount in situ hybridization (Intavis) was performed. Briefly, embryos were progressively re-hydrated, permeabilized by proteinase K (Sigma) treatment before being incubated overnight at 68° C in hybridization buffer containing the MAO probe. After stringent washes, the hybridized probes were detected by immunohistochemistry using an alkaline phosphatase-conjugated antibody against digoxygenin (Roche) and a NBT/BCIP chromogenic substrate (Roche). After staining, embryos and/or brains were dissected out, mounted in glycerol and photographs were taken on a Nikon E800 microscope equipped with a DXM1200 camera. MAO mutagenesis and cell culture assay The pro>leu mouse MAO-A and MAO-B mutant forms were generated from WT- MAOs using site-directed mutagenesis (Quikchange II kit; Stratagene) and sub-cloned in pcDNA3.1 (Invitrogen). COS-7 cells (5 × 10 4 cells per well, 24-well format) were plated in 0.5 ml of complete growth medium. For transfection, cell density was 70~80% confluent. For each well of cells to be transfected, 0.5 μg of DNA was diluted into 100 μl of Opti-MEM medium without serum. Then, 0.5 μl PLUS Reagent (a 1:1 ratio to DNA) was added directly to the diluted DNA and incubated for 15 min at room temperature after a gentle mix. For each well of cells, 2 μl of Lipofectamine LTX was added to the above diluted DNA solution, mixed gently and incubated for 25 min at room temperature. A total of 100 μl of this mixture was added directly to each well and mixed by rocking the plate back and forth. Cells were incubated at 37 °C in a CO 2 incubator for 48 h post transfection before assaying for MAO activity as described above and using tyramine as a substrate. How to cite this article: Elipot, Y. et al. A mutation in the enzyme monoamine oxidase explains part of the Astyanax cavefish behavioural syndrome. Nat. Commun. 5:3647 doi: 10.1038/ncomms4647 (2014).